A polarity-induced defect mechanism for conductivity and magnetism at polar–nonpolar oxide interfaces The discovery of conductivity and magnetism at the polar–nonpolar interfaces of insulating nonmagnetic oxides such as LaAlO 3 and SrTiO 3 has raised prospects for attaining interfacial functionalities absent in the component materials. Yet, the microscopic origin of such emergent phenomena remains unclear, posing obstacles to design of improved functionalities. Here we present first principles calculations of electronic and defect properties of LaAlO 3 /SrTiO 3 interfaces and reveal a unifying mechanism for the origins of both conductivity and magnetism. We demonstrate that the polar discontinuity across the interface triggers thermodynamically the spontaneous formation of certain defects that in turn cancel the polar field induced by the polar discontinuity. The ionization of the spontaneously formed surface oxygen vacancy defects leads to interface conductivity, whereas the unionized Ti-on-Al antisite defects lead to interface magnetism. The proposed mechanism suggests practical design principles for inducing and controlling both conductivity and magnetism at general polar–nonpolar interfaces. Oxide interfaces exhibit many spectacular phenomena not found in the respective bulk components or in conventional semiconductor interfaces [1] , providing new avenues for electronics [2] . The LaAlO 3 /SrTiO 3 interface is a paradigm example, exhibiting conducting two-dimensional (2D) electron gas (2DEG) [3] , [4] and magnetism [5] , [6] , [7] , [8] , [9] , [10] , [11] between two insulating nonmagnetic metal oxides. In the [001] direction, two different interfaces can be formed between polar LaAlO 3 , which consists of alternating LaO) + –(AlO 2 ) − layers, and nonpolar SrTiO 3 , which consists of alternating (SrO) 0 –(TiO 2 ) 0 layers. One is LaO/TiO 2 stacking configuration (so-called n-type) and the other is AlO 2 /SrO configuration (so-called p-type). The remarkable feature is that the conductivity occurs only at n-type interfaces when the LaAlO 3 film thickness ( n LAO ) is larger than three unit cells (uc) [4] , [5] , whereas the magnetism has been observed both at n-type interfaces with n LAO >~3 uc and at insulating p-type interfaces [8] . 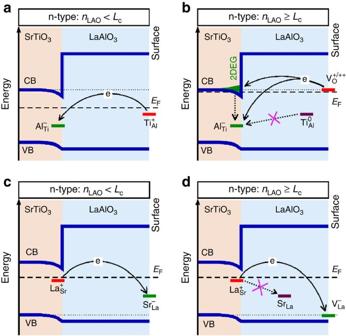Figure 1: Schematic band diagram and change transfer among the defects at LaAlO3/SrTiO3interfaces. (a) n-type interfaces withnLAO<Lc: all electrons transferred from TiAl(S) are trapped by deep AlTi(I), causing no 2DEG. (b) n-type interfaces withnLAO≥Lc:VO(S) defects donate ~0.5e S2D−1to the interface. Part of ~0.5e S2D−1is trapped by the AlTi(I) and the rest leads to interfacial 2DEG. The formed TiAldefects are ionized, i.e., Ti3+-on-Al3+, having local magnetic moments. (c,d) p-type interfaces withnLAO<Lc(~4uc) andnLAO≥Lc: all electrons transferred from LaSr(I) are trapped by SrLa(S) and VLa(S), respectively. All involved defects are deep and do not induce carriers. The un-ionized TiAl0(not shown inc,d) also form and induce local moments. The superscripts (0,+,++,−) in the Figure denote the defect charge states, not the oxidation states of the ions there. Table 1 lists some experimental observations representing the main puzzles [12] that need to be resolved before the promised applications can be realized [13] . Table 1 List of some important experimental observations at LaAlO 3 /SrTiO 3 interfaces. Full size table For 2DEG at n-type interfaces, four main mechanisms have been suggested, yet no single one explains the full scope of these puzzles. The prevalent one is intrinsic electronic reconstruction (so-called polar catastrophe) involving ionization of the electrons from host valence band of LaAlO 3 within the abrupt and defect-free interfaces ( Supplementary Fig. 1 ) [3] , [4] . The other three mechanisms involve various defects, including the oxygen vacancies at the interface (denoted as V O ( I ), where ‘ I ’ means ‘Interface’) [14] , [15] , [16] , oxygen vacancies at LaAlO 3 overlayer surface (denoted as V O ( S ), where S means ‘Surface’) [17] , [18] , [19] , [20] , [21] , [22] , and the La-on-Sr (La Sr ) antisite donor defects induced by interfacial cation intermixing [23] , [24] , [25] , [26] , [27] , [28] , [29] . As Table 1 shows, each of these proposed mechanisms represents one aspect of the interface physics, explains some experimental findings, but conflicts with a few others [2] . None explains the insulating nature of p-type interfaces. Regarding interface magnetism, it was shown experimentally that the local magnetic moments are associated with Ti 3+ ions [5] , [6] , [7] , [8] , [9] , [10] , [11] , [30] . However, it is yet unclear whether such Ti 3+ ions reside in the interface within SrTiO 3 side, or LaAlO 3 side, or both sides. Theoretically, it has been argued that the Ti 3+ ions arise in SrTiO 3 side, owing to the occupation of the low-energy Ti- d xy -like sub-bands caused by the interfacial splitting of orbital degeneracy [31] , or interfacial disorder [32] , [33] , or interfacial oxygen vacancies [34] . However, these scenarios are difficult to explain the fact that magnetism occurs at p-type interfaces and n-type interfaces with a critical thickness ( L c ) similar to that for 2DEG. The centrosymmetric III–III–O 3 perovskite has a non-zero formal polarization, as established by the modern theory of polarization [35] , [36] . The discontinuity in the formal polarization of LaAlO 3 and SrTiO 3 leads to a finite polar field that would cause the divergence of electrostatic potential as the n LAO increases. A crucial issue associated with the emergent conductivity and magnetism at polar–nonpolar interfaces is what mitigates such potential divergence. Is it electronic reconstruction within the polar catastrophe scenario, or the atomic reconstruction scenario with or without chemical defects? Different mechanisms suggest different experimental designs that would control conductivity, mobility and magnetism. Particularly, for defects, it is unclear which defects can be induced and are responsible for the emergent interface phenomena. Using first principles electronic and defect calculations, we find that the certain defects would form spontaneously in response to the built-in polar field. The ensuing polarity-induced defect mechanism ( Fig. 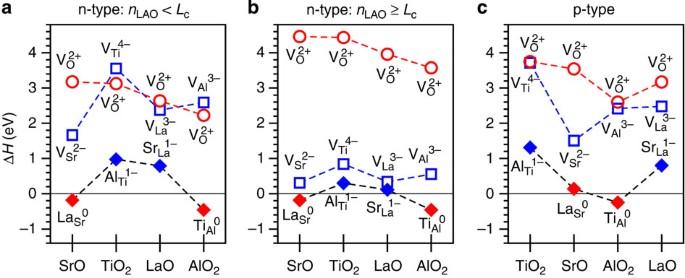Figure 2: Formation energy of the interfacial point defects at thermodynamical equilibrium Fermi energy. (a,b) n-type interfaces with nLAO<LcandnLAO≥Lc, respectively. (c) p-type interfaces. At a givenEF, the defect in different charge states (for example, VSr0, VSr1−, VSr2−) usually has different ΔHand the only one with the lowest ΔHis shown in the Figure. The ΔHversusEFfor these defects are shown inSupplementary Fig. 2, which also includes other high-ΔHdefects not shown here. The chemical potentials used for Sr, Ti, La, Al and O are −4.36, −6.20, −6.10, −5.46 and −2.0 eV, respectively, relative to their corresponding elemental solid or gas phases, which corresponds toT=1050 K andPO2=6.1 × 10−6Torr (Supplementary Fig. 3). 1 ) simultaneously explains the main features of both conductivity and magnetism at the interface, as summarized in Table 2 . Figure 1: Schematic band diagram and change transfer among the defects at LaAlO 3 /SrTiO 3 interfaces. ( a ) n-type interfaces with n LAO < L c : all electrons transferred from Ti Al ( S ) are trapped by deep Al Ti ( I ), causing no 2DEG. ( b ) n-type interfaces with n LAO ≥ L c : V O ( S ) defects donate ~0.5e S 2D −1 to the interface. Part of ~0.5e S 2D −1 is trapped by the Al Ti ( I ) and the rest leads to interfacial 2DEG. The formed Ti Al defects are ionized, i.e., Ti 3+ -on-Al 3+ , having local magnetic moments. ( c , d ) p-type interfaces with n LAO < L c (~4uc) and n LAO ≥ L c : all electrons transferred from La Sr ( I ) are trapped by Sr La ( S ) and V La ( S ), respectively. All involved defects are deep and do not induce carriers. The un-ionized Ti Al 0 (not shown in c , d ) also form and induce local moments. The superscripts (0,+,++,−) in the Figure denote the defect charge states, not the oxidation states of the ions there. Full size image Table 2 The specific defects and their charge transfer processes that explain the leading experimental observations at stoichiometric LaAlO 3 /SrTiO 3 interfaces. Full size table The key defect-related physical quantities that feature in our explanation are (i) the formation energy Δ H of defects in various charge states ( q ) at the thermodynamic equilibrium Fermi energy E F ( Fig. 2 ). This Δ H controls the equilibrium defect concentration; (ii) the defect charge transition energy levels (deep or shallow; Fig. 3 ), ε ( q/q ′) defined as the E F where the Δ H of a defect in two different charge states q and q ′ equal. A donor can produce electrons and compensate holes, whereas an acceptor can produce holes and compensate electrons. These two quantities (i) and (ii) calculated for charged defects located in different layers across the interfaces turn out to be crucial. The details of their first principles calculations are given in the Methods section. Figure 2: Formation energy of the interfacial point defects at thermodynamical equilibrium Fermi energy. ( a , b ) n-type interfaces with n LAO < L c and n LAO ≥ L c , respectively. ( c ) p-type interfaces. At a given E F , the defect in different charge states (for example, V Sr 0 , V Sr 1− , V Sr 2− ) usually has different Δ H and the only one with the lowest Δ H is shown in the Figure. The Δ H versus E F for these defects are shown in Supplementary Fig. 2 , which also includes other high-Δ H defects not shown here. The chemical potentials used for Sr, Ti, La, Al and O are −4.36, −6.20, −6.10, −5.46 and −2.0 eV, respectively, relative to their corresponding elemental solid or gas phases, which corresponds to T =1050 K and P O2 =6.1 × 10 −6 Torr ( Supplementary Fig. 3 ). 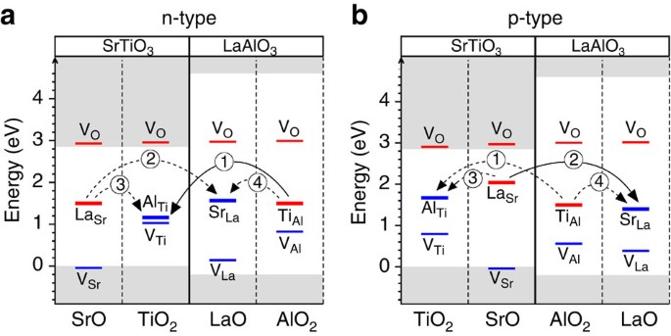Figure 3: Charge transition energy levels of the interfacial point defects. (a) n-type interface. (b) p-type interface. The defect charge transition energy level is defined as theEFwhere the ΔHof a given defect in two different charge states equal. Some defects may have multiple charge transition energy levels. For example, VSrhas the two transition energy levels (one is for the transition between neutral charge state and −1, and the other is between −1 and −2). In such case, if the defect is donor (red), only the lowest level is shown, and if the defect is acceptor (blue), the highest level is shown. Full size image Figure 3: Charge transition energy levels of the interfacial point defects. ( a ) n-type interface. ( b ) p-type interface. The defect charge transition energy level is defined as the E F where the Δ H of a given defect in two different charge states equal. Some defects may have multiple charge transition energy levels. For example, V Sr has the two transition energy levels (one is for the transition between neutral charge state and −1, and the other is between −1 and −2). In such case, if the defect is donor (red), only the lowest level is shown, and if the defect is acceptor (blue), the highest level is shown. Full size image The central point of the proposed mechanism is that the polar-discontinuity-induced built-in polar field triggers thermodynamically the spontaneous formation of certain defects at the surface and/or interface, which in turn compensate the built-in polar field and thus avoids the potential divergence. Thus, it is the polar-field-induced defects, rather than the electronic or atomic reconstruction, that are responsible for the conductivity and magnetism at the interface. Specifically, we find that the surface V O has its donor levels located energetically above the SrTiO 3 conduction band at the interface but below the LaAlO 3 conduction band. This donor level position is a prerequisite for 2DEG formation. Although the occurring of the 2DEG is because of the surface donors, the density of 2DEG is controlled by the interfacial deep acceptor defects (mainly Al-on-Ti antisite). It has also turned out that the interface magnetic moment is caused by the unionized deep Ti-on-Al antisite defects located within the LaAlO 3 side near the interface. We address below how this polar-field-induced defect mechanism resolves the long-standing puzzles on the origin of 2DEG, the critical thickness for 2DEG, the weak field in LaAlO 3 film, the density of 2DEG, the insulating nature of p-type interfaces and the origin of the local magnetic moments. During this process, we also distil the general design principles that control the pertinent effects and could allow future section of better polar–nonpolar interface materials. The origin of the 2DEG The 2DEG is unlikely to originate from the defect-free scenarios: these include the ionization of the intrinsic LaAlO 3 valence bands (suggested by the polar catastrophe model [3] , [4] ) or the ionization of the LaO interface layer (suggested by the interfacial charge-leaking model) [37] ( Supplementary Note 1 ). This conclusion stems from the fact that the creation of 2DEG in these defect-free scenarios requires the LaAlO 3 valence band maximum (VBM) to cross the SrTiO 3 conduction band minimum (CBM) or E F . However, this is contrary to the experimentally observed weak field (negligible band-bending) [38] , [39] , [40] , [41] in the LaAlO 3 film, clearly showing that the LaAlO 3 VBM is located energetically far below the E F . The 2DEG also is unlikely to originate from interfacial point donor defects (La Sr , Ti Al and V O ). Recall first that the defect formation energy (Δ H ) depends on the E F (or chemical potential) and the defect charge transition energy ε ( q/q ′) needs to be close to band edges in order to produce free carriers. In thermodynamic equilibrium, the E F of the system pins around the middle of SrTiO 3 band gap when n LAO < L c and around the SrTiO 3 conduction band edge near the interface when n LAO ≥ L c ( Supplementary Note 2 ). In either case, Fig. 2ab shows that the Δ H of the interfacial antisite donor defects, La Sr 0 and Ti Al 0 , is small positive or even negative (note: the superscript denotes the defect charge states, not the nominal oxidation state of the atom at the defect site). In other words, the formation of such antisite defects at the thermodynamic equilibrium E F is energetically favourable and would inevitably lead to interfacial cation mixing. However, at such E F , both La Sr 0 and Ti Al 0 defects are stable in their charge neutral states (as indicated by the superscript), contributing no free carriers. On the other hand, the interfacial V O defects are energetically stable in the charged states, that is, V O 2+ ( Fig. 2a,b ). This means that, if formed, the V O will donate electrons and thereby become positively charged. However, the Δ H of V O 2+ at such equilibrium E F is rather high (>2.5 eV), implying that V O 2+ have very low concentration under thermodynamic equilibrium conditions. The high Δ H also means that even if the V O defects are formed under nonequilibrium growth conditions, they can still be removed easily by the post O-rich annealing process [42] ( Supplementary Note 3 ). Thus, contrary to earlier postulations, these interfacial donor defects are not responsible for 2DEG, consistent with recent experiments [43] . The oxygen vacancy, V O ( S ), at the free LaAlO 3 surface can explain the interfacial 2DEG. For this to happen, three conditions (‘design principles’) need to be satisfied. First, V O ( S ) in the polar film material needs to have a sufficiently low formation energy Δ H ; therefore, it could form in significant quantities. 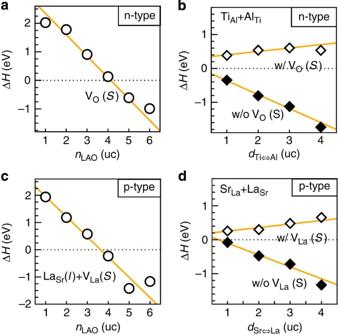Figure 4: Properties of surface defects and defect complexes. (a) The GGA-calculated ΔHof VO(S) defect, under the O-rich growth condition (that is, ΔμO=−1.5 eV,Supplementary Fig. 3a). (b) the ΔHof [TiAl+AlTi] defect pair created from a Ti⇔Al exchange out of the ideal interface with and without a VO(S) in a 2 × 2 (SrTiO3)6/(LaAlO3)4/vacuum surpercell. (c) The GGA-calculated ΔHof [LaSr(I)+VLa(S)] defect complex as a function ofnLAO, under ΔμSr=−4.36 eV (Supplementary Fig. 3b). (d) the ΔHof [LaSr+SrLa] defect pair created from a La⇔Sr exchange out of the ideal interface with and without a VLa(S) in a 2 × 2 (SrTiO3)6/(LaAlO3)4/vacuum surpercell, respectively. ThedTi⇔AlanddLa⇔Srinb,dare the distance between the components of corresponding defect pair. The orange lines are the guides to the eye. Figure 4a shows that the Δ H of V O ( S ) decreases linearly as the film thickness n LAO increases, consistent with previous calculations [20] , [44] . When n LAO ≥3–4 uc, the Δ H becomes zero or negative, and V O ( S ) will form spontaneously. The large negative Δ H means that even exposing the surface to air or post annealing under O-rich environment cannot remove these vacancies. Second, the system needs to have a none-zero built-in polar field that would enable the electron to transfer from the surface of the polar material to the interface. Such transfer sets up an opposite dipole (proportional to n LAO ), which in turn cancels the field and lowers the Δ H . The larger the n LAO , the lower the Δ H . Note that in the absence of such field, the surface-to-interface charge transfer would not occur since such a transfer would create a dipole that would increase the electrostatic energy (proportional to that dipole) and thus raise the total energy of the system. Third, the donor transition level of V O ( S ) in the polar film should be higher in energy than in the substrate (SrTiO 3 ) conduction band edge at the interface ( Fig. 3 ). These three conditions are satisfied in this LaAlO 3 /SrTiO 3 system. Figure 4: Properties of surface defects and defect complexes. ( a ) The GGA-calculated Δ H of V O ( S ) defect, under the O-rich growth condition (that is, Δ μ O =−1.5 eV, Supplementary Fig. 3a ). ( b ) the Δ H of [Ti Al +Al Ti ] defect pair created from a Ti ⇔ Al exchange out of the ideal interface with and without a V O ( S ) in a 2 × 2 (SrTiO 3 ) 6 /(LaAlO 3 ) 4 /vacuum surpercell. ( c ) The GGA-calculated Δ H of [La Sr ( I )+V La ( S )] defect complex as a function of n LAO , under Δ μ Sr =−4.36 eV ( Supplementary Fig. 3b ). ( d ) the Δ H of [La Sr +Sr La ] defect pair created from a La ⇔ Sr exchange out of the ideal interface with and without a V La ( S ) in a 2 × 2 (SrTiO 3 ) 6 /(LaAlO 3 ) 4 /vacuum surpercell, respectively. The d Ti ⇔ Al and d La ⇔ Sr in b , d are the distance between the components of corresponding defect pair. The orange lines are the guides to the eye. Full size image It is noteworthy that it is the built-in polar field that triggers the spontaneous formation of the V O ( S ) when n LAO ≥ L c . Such built-in polar field always exists in the LaAlO 3 to be grown during the layer-by-layer growth. This is because that the surface defects (here V O ) can cancel the built-in polar field only in the LaAlO 3 film between the interface and the surface, not the built-in polar field in the LaAlO 3 film to be grown on top of the surface. In the absence of interfacial defects, the emerging picture for creating 2DEG is that the electrons ionized from V O ( S ) of the polar film material transfer to the nonpolar substrate material SrTiO 3 conduction bands at the interface via the built-in polar field, thus forming the 2DEG at that interface. This charge transfer in turn cancels the built-in polar field in LaAlO 3 , which caused the low Δ H of the surface vacancies in the first place. After the built-in field has been cancelled, the Δ H of V O ( S ) return to a high value (>3 eV) characteristic of the bulk, and V O ( S ) become again hard to form in thermodynamic equilibrium [20] . Thus, the theoretical maximum concentration of V O ( S ) is 0.25 S 2D −1 (where S 2D is 2D unit cell area), that is, one of eight oxygen missing at surface. These would donate maximally 0.5e S 2D −1 that would completely cancel the polar field in LaAlO 3 . The compensation of polar field by V O ( S ) also means that the band bending in LaAlO 3 because of polar field is removed. Thus, the LaAlO 3 valence bands fall well below the E F , contrary to what the polar catastrophe model would suggest. Consequently, no free holes can arise from depopulation of the LaAlO 3 valence bands at the surface, consistent with experiments [3] , [22] . The emerging design principles for selecting materials that will form interfacial 2DEG are: (i) the nonpolar material needs to have a CBM positioned in the band gap of the polar material; (ii) the polar material needs to have at least one donor defect with its donor level higher in energy than the conduction band of the nonpolar material at the interface. This picture suggests that the 2DEG at n-type LaAlO 3 /SrTiO 3 interfaces may also be induced and/or tuned by using certain surface adsorbates (for example, H 2 O and H) [45] , [46] , [47] or metallic contacts [48] provided that the ionization energy of the surface adsorbate or the metallic contact is not lower than the donor level of the V O ( S ). The origin of the critical thickness The linear decrease in ΔH of V O ( S ) with increasing polar film thickness n LAO naturally explains the critical thickness L c for the metal–insulator transition. The calculated rate of decrease (that is, the slope dΔ H/ d n LAO ) equals 0.19 eV Å −1 , which is the same as the calculated built-in polar field in the defect-free LaAlO 3 film ( Supplementary Note 4 ). The V O ( S ) defects start to form spontaneously when the Δ H becomes zero at the L c of ~4 uc under a typical O-rich growth condition ( Fig. 4a ). For the LaAlO 3 film that is 1 uc thinner than this L c , the calculated Δ H of V O ( S ) is 0.75 eV, which is too high to produce significant free carrier concentration. Thus, the appearance of V O ( S ) (and the ensuing metal–insulator transition) at L c is predicted to be a sharp transition ( Supplementary Note 5 ), distinct from the gradual appearance of 2DEG behaviour as predicted from polar catastrophe model, but consistent with experiments [49] . Figure 3a suggests that the L c resulting from V O ( S ) can be written as L c =Δ H o /eE p , where Δ H o is the formation energy of the V O at interface (or the Δ H extrapolated at n LAO =0) and E p is the built-in polar field. Using E p =4 πP 0 / ε (where ε and P 0 are the dielectric constant and formal polarization of LaAlO 3 film), this relation can be written as which predicts an L c of ~4 uc, depending slightly on the O-poor/rich growth conditions ( Supplementary Note 6 ). The above formula provides an alternative explanation for the observed variation of the L c with the fraction x in (LaAlO 3 ) 1− x (SrTiO 3 ) x overlayer (where P 0 is proportional to x ) [50] . This observation was originally explained by L c =Δ Φε /4 πeP 0 (where Δ Φ is the energy difference between LaAlO 3 VBM and SrTiO 3 CBM) within polar catastrophe model [50] . Since Δ Φ and Δ H o have accidentally similar value (~3–4 eV) in this system, it is not surprising that the L c predicted from these two models is also similar. However, the V O ( S ) model clearly explains many other observations in which the polar catastrophe model fails ( Table 1 ). Implication on the design of carrier mobility: (i) the relatively high 2DEG mobility could be enabled by a modulated doping effect [51] , whereby the source of carriers (here at the LaAlO 3 surface) is spatially separated from the location where the carriers reside (here at the LaAlO 3 /SrTiO 3 interface), thus minimizing carrier scattering by the ionized defects. This minimal spatial separation is measured by the critical thickness L c . The equation (1) suggests that a large L c (hence maintaining good mobility) could be achieved by selecting a polar materials with small polarization, large dielectric constant and donor defects having high Δ H at the interface or in the bulk. On the other hand, (ii) the concentration of interfacial defects must be minimized in order to take advantage of (i). In addition, (iii) since the 2DEG is located at the conduction bands of the nonpolar material, it is advantageous to select the nonpolar material with low electron effective mass in order to achieve higher mobility. Polar field compensation Experimentally, only very weak residual field has been observed in the LaAlO 3 film no matter whether its thickness is below or above the L c (refs 38 , 39 , 40 , 41 , 52 ). This observation cannot be explained within the defect-free interface scenario, even including the ionic relaxations [53] . In turn, whereas the V O ( S ) model explains the weak electric field in LaAlO 3 film above the L c , it does not explain it below the L c . This leads us to inspect the effects of all possible cation antisite defects across the interface. Each individual interfacial antisite alone cannot cancel the polar field. Figure 2ab shows that the La Sr , Sr La , Ti Al and Al Ti antisite defects have lower Δ H than other point defects (for example, cation vacancies) in the layer where they are located. Therefore, the former are the dominant defects in their corresponding layers. The interfacial La Sr donor in the SrTiO 3 side cannot set up an opposite dipole across the LaAlO 3 film that can cancel the polar field inside the LaAlO 3 film. Regarding the Ti Al donor in the LaAlO 3 side, the donor level is lower than the SrTiO 3 conduction band at the interface. Therefore, the ionized electrons cannot be transferred to the latter so as to cancel the polar field. Regarding the interfacial Al Ti and Sr La acceptors, the polar field compensation is similar to that in the polar catastrophe model: before the LaAlO 3 VBM reaches the acceptor levels of Al Ti or Sr La , the polar field cannot be cancelled. The [Ti Al +Al Ti ] defect pair is the most potent source of polar field cancellation among those donor–acceptor antisite defect pairs at n-type interfaces. The four leading antisite defects can form four types of donor–acceptor pairs: [Ti Al +Al Ti ], [La Sr +Sr La ], [La Sr +Al Ti ] and [Ti Al +Sr La ], denoted as , , and , respectively, in Fig. 3 . Clearly, the electron transfer from donor to acceptor in both pairs and is unlikely since it will create a dipole in the same direction as the intrinsic dipole in LaAlO 3 , and thus increase the dipole moment (also the electrostatic energy) and destabilize the interface. In pairs and , the charge transfer can cancel the polar field. However, the electron transfer in pair is energetically much more favourable because, first, Al Ti has a lower acceptor level than Sr La and, second, the donor–acceptor separation distance (also the associated opposite dipole moment that lowers the total energy of the system) is larger in pair ( Fig. 3a ). We thus next focus on [Ti Al +Al Ti ] (that is, pair ). For n LAO < L c , the [Al Ti +Ti Al ] antisite pair can form spontaneously via Ti ⇔ Al exchange across the interface and cancel the polar field. Figure 4b (filled symbols) shows that the energy required to form such defect pair is negative (that is, exothermic), and the largest energy gain is obtained when a Ti atom of TiO 2 -interface monolayer is exchanged with an Al of AlO 2 -surface monolayer, that is, Al Ti ( I )+Ti Al ( S ), which is consistent with previous first principles calculations [54] . This means that Ti atom at the interface would hop to the AlO 2 -surface layer and exchange with Al atom there. Similar to the case of V O ( S ), the linear decrease in Δ H with increasing donor–acceptor separating distance ( Fig. 4b ) is a sign of polar field compensation. Indeed, the electron transfer from the Ti Al donor to the Al Ti acceptor is expected, since the donor level is higher in energy than the acceptor level ( Fig. 3a ). Figure 4a also shows that the V O ( S ) has too high Δ H to form for n LAO < L c ( Fig. 4a ). Therefore, the polar field is cancelled by those spontaneously formed [Al Ti ( I )+Ti Al ( S )] pairs. On the other hand, since these defects are deep, they cannot cause free carriers in the both interface and surface regions (whence insulating). For n LAO ≥ L c , the polar field is cancelled by spontaneously formed V O ( S ), not by [Al Ti (I)+Ti Al (S)]. Recall that the polar field always exists in the LaAlO 3 layers during the layer-by-layer growth. Such polar field can trigger the formation of V O ( S ) and/or Ti Al ( S ) defects as n LAO increases. For n LAO ≥ L c , both V O ( S ) ( Fig. 4a ) and [Al Ti ( I )+Ti Al ( S )] pair ( Fig. 4b ) have zero or negative Δ H , meaning that both could form in ideal interfaces. However, if both V O ( S ) and Ti Al ( S ) are present, since V O has an energetically higher donor level than Ti Al ( Fig. 3a ), the V O ( S ) would transfer electrons to the Ti Al defects. The polar field that was initially cancelled by the electrons transferred from the Ti Al defects are then released and get cancelled by the electrons transferred from V O ( S ) defects. Consequently, the polar field in the whole LaAlO 3 film would be cancelled by the V O ( S ) defects (if present). The larger the n LAO , the lower the Δ H of the V O ( S ). After the polar field has been cancelled by V O ( S ), Fig. 4b (open symbols) shows that the Δ H of [Al Ti ( I )+Ti Al ( S )] pair becomes positive (0.4–0.7 eV), meaning that [Ti Al +Al Ti ] pairs cannot be formed via Ti ⇔ Al exchange over a distance beyond L c . In brief, the presence of the [Ti Al +Al Ti ] defect pairs in the sample does not change the linear-decreasing behaviour in the Δ H of the V O ( S ) ( Fig. 4a ), suggesting that the metal–insulator transition still occurs at the L c of ~4 uc. However, the presence of V O ( S ) would prevent [Ti Al +Al Ti ] pairs forming further above the L c , and reduce the concentration of these pairs formed below the L c . The density of the 2DEG Reinterpretation of the puzzle: According to Gauss’ law, the experimentally observed weak electric field in LaAlO 3 film means that the total external charge density (mobile and/or immobile) at the interface must be ~0.5e S 2D −1 ( Supplementary Note 7 ), as recently observed [55] . For n LAO < L c , there is no interfacial conductivity and thus none of these interfacial charge contribute to the conductivity. For n LAO ≥ L c , only a fraction of 0.5e S 2D −1 interfacial charge is seen in transport, and so the majority of 0.5e S 2D −1 charges do not contribute to the conductivity. The puzzle thus is why the ~0.5e S 2D −1 charge exists at the interface with any n LAO , but only a small part of it contributes to conducting 2DEG when n LAO ≥ L c . This puzzle cannot be explained by defect-free polar catastrophe model [3] , [4] or interfacial charge-leaking model [37] , since both predict zero interfacial charge for n LAO < L c and an interfacial charge density much higher than the measured 2DEG density for n LAO ≥ L c ( Supplementary Fig. 1 ). The possibility of ‘multiple carrier types’ at defect-free interfaces (that is, those electrons occupying interfacial d xy sub-band and those occupying d xz / d yz sub-bands contribute differently in transport) has also been suggested to explain the measured 2DEG density above the L c (refs 56 , 57 , 58 , 59 ). However, this scenario could not explain the total 0.5e S 2D −1 interface charge that is independent of n LAO . Moreover, it is also difficult to explain why a full carrier density of 0.5e S 2D −1 has been observed at GdTiO 3 /SrTiO 3 interfaces (where the same multiple carrier types exist) [60] . The 2DEG density is controlled by the concentration of immobile acceptor defects that can trap itinerant electrons. Within the emerging defect picture, the total interfacial charge is always ~0.5e S 2D −1 , which corresponds to the (almost) complete polar field cancellation. In the SrTiO 3 side (where the 2DEG is located), there are mainly three types of acceptor defects, namely, Al Ti , V Sr and V Ti . At equilibrium E F , Fig. 2a,b shows that these acceptor defects all prefer to stay in negative charge states, that is, Al Ti 1− , V Sr 2− and V Ti 4− . (In other defect charge states, these defects have much higher Δ H and are not shown in Fig. 2a,b . ). This means that once these defects form they will trap free electrons from the system and get negatively charged. Among these acceptor defects, the Al Ti 1− acceptors have the lowest Δ H and thus they the most potent electron-trapping agents. For n LAO < L c , the Al Ti defects resulting from Ti ⇔ Al exchange trap all free electrons transferred from Ti Al ( S ) defects, and hence no free carrier can occur. For n LAO ≥ L c , the Δ H of [Ti Al +Al Ti ] pair changes from negative to positive because of V O ( S ) ( Fig. 4b ), meaning that the concentration of Al Ti defect resulting from Ti ⇔ Al exchange is reduced, compared with that formed below the L c . Therefore, the Al Ti defect concentration is not sufficient to trap all 0.5e S 2D −1 electrons transferred from V O ( S ). Therefore, only a small fraction of 0.5e S 2D −1 can contribute to interface 2DEG. The recently observed LaAlO 3 cation-stoichiometry effect on 2DEG formation [43] may also be understood within the above picture. For Al-rich LaAlO 3 film, where both A-site and B-site sublattices are fully occupied (hence having no cation vacancies), the Al Ti antisites are the only electron-trapping defects and the incomplete trapping of 0.5e S 2D −1 interface charge by Al Ti defects leads to interface conductivity. However, for La-rich LaAlO 3 film, where B-site sublattice is not fully occupied, the cation vacancies (V Ti and V Al ) also become the main electron-trapping agents, in addition to Al Ti ( I ). Although the concentration of Al Ti is reduced, each cation vacancy induced in the La-rich film traps more electrons than an Al Ti . The insulating character can thus be then attributed to the complete interfacial electron trapping by both interfacial cation vacancies and Al Ti ( I ). The picture of Al Ti ( I ) as the main electron-trapping agent may be extended to SrTiO 3 /GdTiO 3 interfaces. The observed full carrier density of 0.5e S 2D −1 there [60] can be ascribed to the fact that both SrTiO 3 and GdTiO 3 have the same Ti atom at B-site sublattice and thus have no Al Ti -like antisite defects at the interface. Implication on how to increase the density of 2DEG: The above picture suggests that the main controlling factor for the interface carrier density is the concentration of the acceptor defects (mainly Al Ti in stoichiometric or Al-rich film), which should be minimized for enhancing carrier density. Such Al Ti -like electron-trapping defects may be completely removed by designing other oxide interfaces such as GdTiO 3 /SrTiO 3 interfaces, whose bulk components have a common cation atom with multiple valence states. The origin of the insulting nature of p-type interfaces An intriguing fact is that the so-called p-type interfaces are not p-type (hole) conducting but are actually insulating. The defect-free polar-catastrophe model for p-type interface predicts a hole-conducting interface and an electron-conducting surface when n LAO >~ 7.3 uc ( Supplementary Fig. 1 ) in contradiction with the insulating behaviour observed robustly in experiment. To explain this, defects must be involved. The emerging defect picture below differs from the literature model based solely on interfacial hole–polaron [61] or interfacial hole-compensating V O defects [23] , [44] , which assumes that the interface has holes arising from the depopulation of the intrinsic SrTiO 3 valence bands. Individual point defects alone at p-type interfaces can neither cause conductivity nor cancel the polar field. As was the case for n-type interfaces, Fig. 2b shows that the interfacial La Sr and Ti Ar are stable at their charge neutral states and have negligible or negative Δ H at equilibrium E F . This means that they cause inevitable interfacial cation intermixing but induce no free carriers. The V O and other defects at the interface require too high Δ H to form, and thus they do not produce free carriers either. For similar reason, each of the leading antisite defects (La Sr , Sr La , Ti Al and Al Ti ) alone at p-type interfaces cannot cancel the polar field. The spontaneously formed donor–acceptor defect pairs always cancel the polar field but do not induce free carriers. Among the four donor–acceptor defect pairs as indicted in Fig. 3b , the [La Sr +Sr La ] (that is, pair ) is energetically most favourable to cause polar field cancellation. For n LAO <~ 4 uc, the [La Sr ( I )+Sr La ( S )] pairs have negative Δ H ( Fig. 4d ) and can form spontaneously via La ⇔ Sr exchanges, whereas the [La Sr ( I )+V La ( S )] have too high Δ H to form ( Fig. 4c ). Therefore, the polar field is cancelled by the charge transfer from La Sr ( I ) to Sr La ( S ), which can be expected from their relative defect levels ( Fig. 3b ) and their linear decreasing behaviour in Δ H as a function of n LAO ( Fig. 4d ). For n LAO ≥~4 uc, the Δ H of [La Sr ( I )+V La (S)] become negative ( Fig. 4c ) and can also form spontaneously. Since V La has a lower acceptor level than Sr La ( Fig. 3b ), the polar field is cancelled by the charge transfer from La Sr ( I ) to V La ( S ), rather than to Sr La ( S ). In absence of an electric field, Fig. 4d (open symbols) indicates that the La ⇔ Sr exchanges cannot occur anymore over a distance of ~4 uc. Unlike the case in n-type interfaces, the V O ( S ) defects in p-type interface always have too high Δ H to form. The defects involved in polar field cancellation are all deep. The calculated equilibrium E F according to those point defects turns out to be always around the middle of SrTiO 3 band gap. This means that both VBM and CBM are far away from the E F , and there are no free carrier arising from the depopulation of VBM and CBM in both interface and surface regions (whence insulating). Implication on the design of 2D hole conductivity: Clearly, the formation of interfacial free holes is prevented by these spontaneously formed deep La Sr defects that have donor level higher than the VBM at the interface. Therefore, to induce interfacial hole conductivity, one should search for the polar–nonpolar interfaces where all such donors have high enough formation energy to form or (ii) their donor levels below the VBM at the interface. Practically, the (ii) may be achieved more easily by searching for the polar material whose VBM is higher than the charge transition energy levels of those spontaneously formed interfacial donor defects. The origin of interface magnetism Distinct from previous models [31] , [32] , [33] , [34] that explain magnetism based on the intrinsic interfacial Ti 3+ ion in the SrTiO 3 (that is, not a defect), we find below that the local magnetic moment originates from the unionized deep Ti Al antisite defect (that is, Ti 3+ -on-Al 3+ within LaAlO 3 side near the interface. The interface magnetism depends on the concentration and spatial distribution of such Ti Al defects. This picture explains not only why the magnetism appears at n-type interfaces with a similar critical thickness to that for 2DEG but also why the magnetism also appears at insulating p-type interfaces [8] . What causes local moment? As discussed earlier, for n-type interfaces, when n LAO < L c , the polar field in LaAlO 3 is cancelled by the charge transfer from Ti Al ( S ) defects to the interface. These formed Ti Al defects are thus ionized, that is, Ti Al 1+ (where superscript denotes the defect charge states). The Ti ion at this defect site has the oxidation states of 4+, denoted as Ti 4+ , which has no local magnetic moment. Moreover, noted before, when n LAO ≥ L c , the polar field in LaAlO 3 is cancelled by the charge transfer to the interface from V O ( S ) instead of Ti Al . In absence of internal field, all Ti Al ( I ) defects in the LaAlO 3 film are most stable in their charge neutral (or unionized) states, that is, Ti Al 0 , where Ti appears as Ti 3+ oxidation state, having a finite local magnetic moment. Therefore, the interface magnetism at n-type interfaces because of those unionized Ti Al 0 defects should also have a critical thickness of ~4 uc. For p-type interfaces, it is the charge transfer among the defects other than Ti Al defects that cancels the polar field in LaAlO 3 . Thus, all Ti Al defects formed there are not ionized, having local magnetic moments, and cause interface magnetism. The magnitude of local magnetic moment: The local moment of a single Ti Al defect at the interface can be estimated from that in bulk LaAlO 3 , which is 0.84 μ B from our hybrid functional calculation. For ferromagnetic order as observed in the experiment, the total interface magnetic moment depends on the concentration of unionized Ti Al defects in LaAlO 3 and can be very small per Ti atom in average. The experimentally observed inhomogeneous landscape of magnetism that also varies from sample to sample [8] , [9] may be attributed to the various spatial distributions of Ti Al defects, which may be sensitive to sample preparation conditions (such as temperature and P O2 ) and local strain. The Ti Al ( I ) defects within LaAlO side being the origin of the local moment are more reasonable than V O ( I ) in two aspects. First, the deep Ti Al defect is spatially localized and has an unambiguous local moment. In contrast, V O is a shallow donor that transfer electrons to the lower-energy interfacial Ti d xy sub-bands that have light effective mass inside the interface plane [59] ; therefore, the resulting Ti 3+ may then be itinerant. Second, the Ti Al defects would form readily because of the small or negative Δ H of Ti Al , whereas the interfacial V O requires significant energy to form and if formed it may be removed completely after annealing. We establish a physical link between polar discontinuity and defect formation: the polar discontinuity triggers spontaneous formation of certain defects that in turn cancel the polar field induced by polar discontinuity. It is the subtle interplay of those spontaneously formed surface vacancy defects and interfacial cation antisite defects that control the physics of the system by their formation energies and relative defect levels. Table 2 summarizes how those defects shown in Fig. 1 explain the leading experimental observations and puzzles in Table 1 . The explanation leads to a set of design principles for both conductivity and magnetism at LaAlO 3 /SrTiO 3 and other polar–nonpolar interfaces and enables the design of better polar–nonpolar interfaces. Having ruled out the electronic reconstruction, interfacial V O and interfacial cation intermixing mechanism as the possible origin of 2DEG in our calculations, we conclude that the 2DEG at n-type interfaces with n LAO ≥ L c originates from the spontaneously formed V O (S) defects. This conclusion stems from the finding that the donor level of deep V O in the LaAlO 3 side is higher than the SrTiO 3 conduction band edge at the interface. This finding explains why the formation energy of V O (S) decreases linearly as n LAO increases. This linear decrease relation leads to some new controlling parameters for the critical thickness of sharp metal–insulator transition in absence of the electric field in the polar LaAlO 3 film. Instead of causing the 2DEG, the anti site defect pair turns out to play a key role in canceling the polar field, controlling the density of the 2DEG, and inducing the local magnetic moments at the interface ( Table 2 ). The emerging mechanism provides three distinctive predictions to be tested in experiment as further validation. (i) For n-type interfaces, the AlO 2 -surface layer is dominated by Ti Al defects when n LAO < L c and by V O defect when n LAO ≥ L c . (ii) For p-type interfaces, the LaO-surface layer is dominated by Sr La and V La defects, respectively, below and above an L c of ~4 uc. (iii) Ti 4+ and Ti 3+ signals exist in both sides of the interface. The appearance of the Ti 3+ signals should not be taken as a sign of conductivity. Whether the Ti 3+ signals detected by photoemission below the L c (refs 21 , 40 , 62 , 63 ) can be truly assigned to those Ti 3+ ions in the SrTiO 3 side should be revisited carefully. How these Ti Al local moments are ordered (ferromagnetic, or antiferromagnetic, or else) and whether and how they interact with the itinerant 2DEG are still open questions that should be investigated further. Computational techniques All calculations were performed using density functional theory and plane-wave projector-augmented wave [64] method as implemented in the VASP code [65] . An energy cutoff of 400 eV was used. The Brillouin zone was sampled by 8 × 8 × 1 and 4 × 4 × 1 k -point mesh for 1 × 1 and 2 × 2 in-plane supercell, respectively. The atomic forces were relaxed to be less than 0.03 eV Å −1 . The in-plane lattice constant was fixed to 3.943 Å (the relaxed lattice constant of SrTiO 3 by GGA [66] ). In slab calculations, the 4-uc (~16 Å) vacuum layer was used and the dipole correction was always applied to remove artificial dipole interactions [67] . The results in Figs 2 and 3 were obtained by using HSE hybrid functional [68] on top of the GGA-relaxed structures. First principles defect theory The formation energy of a defect (D) calculated from , where and are the total energies of a supercell with and without defect, respectively, and D is in charge state q . n α is the number of atoms of species α needed to create a defect. E F is the Fermi energy relative to VBM ( E v ). Δ μ α is the relative chemical potential of species α with respect to its elemental solid (gas; μ 0 ). The equilibrium Fermi energy was calculated self-consistently according to charge neutrality condition [69] . The chemical potentials relative to their elemental solid (or gas) phase are taken as variables and are bounded by the values that maintain a stable host compound and avoid the formation of other competing phases in thermodynamic equilibrium ( Supplementary Fig. 3 ). The details of theory and calculations can be found in ref. 70 . How to cite this article: Yu, L. et al. A polarity-induced defect mechanism for conductivity and magnetism at polar–nonpolar oxide interfaces. Nat. Commun. 5:5118 doi: 10.1038/ncomms6118 (2014).